Narrowband light detection via internal quantum efficiency manipulation of organic photodiodes Spectrally selective light detection is vital for full-colour and near-infrared (NIR) imaging and machine vision. This is not possible with traditional broadband-absorbing inorganic semiconductors without input filtering, and is yet to be achieved for narrowband absorbing organic semiconductors. We demonstrate the first sub-100 nm full-width-at-half-maximum visible-blind red and NIR photodetectors with state-of-the-art performance across critical response metrics. These devices are based on organic photodiodes with optically thick junctions. Paradoxically, we use broadband-absorbing organic semiconductors and utilize the electro-optical properties of the junction to create the narrowest NIR-band photoresponses yet demonstrated. In this context, these photodiodes outperform the encumbent technology (input filtered inorganic semiconductor diodes) and emerging technologies such as narrow absorber organic semiconductors or quantum nanocrystals. The design concept allows for response tuning and is generic for other spectral windows. Furthermore, it is material-agnostic and applicable to other disordered and polycrystalline semiconductors. Photodiodes are the most common photodetector architecture and are generally classified as broadband (panchromatic) or narrowband (wavelength selective), depending on their spectral responsivity bandwidth [1] . In general, for broadband systems it is desirable to have a spectrally flat, high external quantum efficiency (EQE) across the wavelength range of interest [2] . Broadband photodiodes are used predominantly in multi-colour photodetection under low light conditions (for example, in day-or-night surveillance)—essentially operating as integrating detectors. For narrowband applications such as full-colour imaging or visible-blind near-infrared (NIR) detection (for example in light curtains, security systems and intelligent monitoring), spectral (colour) discrimination is required. This can be achieved with one of two possible approaches: the use of a broadband detector in combination with a dichroic prism or set of optical filters at the input side (we refer to this as input filtering); or the use of a truly narrowband detector with photoresponsive semiconductors engineered for the desired spectral window. The former option has been the predominant strategy for inorganic semiconductor-based narrowband photodetection [3] . However, such a strategy complicates the design of the image sensor and can also lead to degradation of the picture quality and colour constancy [4] , [5] , [6] , [7] , [8] . The molecular nature of organic semiconductors means that organic photodiodes (OPDs) can be designed with relatively narrow spectral responses of <200 nm full-width-at-half-maximum (FWHM) and respectable EQEs (10–30%), but the suppression of response outside the chosen spectral window still remains a significant constraint [8] . For certain imaging applications such as machine vision systems, the ideal case is a quasi-Gaussian spectral response with a FWHM≤100 nm that does not give a response (that is, ‘blind’) outside the chosen window [9] . There is growing interest in the development of new materials and OPD architectures that selectively detect light in the red (620–750 nm) or NIR [2] , [10] . Red light photodetectors are useful for short-distance optical communications [11] and they also form a critical component in three-and-four-colour photosensors [9] , [12] . The best examples have FWHMs of ~200 nm but with significant and undesirable blue and green sensitivity [8] , [13] , [14] . NIR photodetectors are important in medical, industrial, communication, scientific and military applications as well as for night-vision imaging and security [14] , [15] , [16] . NIR-sensitive photodectectors have previously been demonstrated using inorganic quantum dot sensitization [17] , [18] , narrow optical-gap donor organic semiconductors within a conventional thin heterojunction structure [14] , [19] , [20] , and more recently by harvesting sub-gap charge transfer states (CT) [15] , [21] , [22] . Yang et al. have reported on the use of CT state absorption to extend the spectral response of an OPD based on a P3HT:PC60BM blend to the NIR [22] . It is important to note that this is not a particularly efficient method to produce a NIR response since the CT state absorption is very weak in organic semiconductors [21] and therefore extremely thick junctions (>10 μm) are required for light harvesting via CT states. As a consequence, the OPDs of Yang et al. [22] could only be operated at extremely large reverse bias voltages (>100 V), and they also had a very high dark current noise. A truly narrowband (FWHM<100 nm), low noise, visible-blind NIR detector is yet to be realized. The aforementioned thin heterojunction architecture has become the standard design for OPDs. The heterojunction contains two components: an electron acceptor and electron donor, akin to n - and p -type inorganic semiconductors, respectively. The acceptor and donor are either blended at the molecular scale to form a bulk heterojunction (BHJ) [23] or deposited sequentially to form a planar heterojunction [24] . In both cases the photo-active junction is typically of the order 10 to 100 nm in thickness, and is sandwiched between anode and cathode electrodes (one of which is semi-transparent) and various blocking or transport layers. In these heterojunctions, careful attention must be given to the optical absorption of the acceptor and donor since both can contribute to the photocurrent through the so-called photo-induced electron (Channel I) and hole transfer (Channel II) processes [25] . While a large range of electron donor materials are available [6] , [8] , [15] , [19] , the choice of electron acceptor is somewhat limited and is dominated by the fullerenes such as PC60BM ([6,6]-phenyl-C 60 -butyric acid methyl ester) and PC70BM ([6,6]-phenyl-C 70 -butyric acid methyl ester). [1] A relatively small number of non-fullerene acceptors have been reported but very few exhibit acceptable quantum efficiencies within organic photovoltaic cells [26] . This is problematic for narrowband red or NIR OPDs since the fullerenes all possess significant blue–green absorption—considerably broadening the overall device response and/or rendering the detector non-blind in the visible [14] , [27] . The best narrowband red and NIR OPDs to date are based on engineering the absorption spectrum of the materials, rather than a broadband junction plus filter or prism designs [8] , [28] . Conventional heterojunction OPDs are thin film, low finesse cavities [29] . As such, the EQE of the diode is dictated by the absorption of the junction components modified by interference effects derived from multiple reflections between the metallic and semi-transparent electrodes. These micro-cavity phenomena can act to broaden or narrow certain spectral features [30] . Understanding this physics provides additional tools for response tuning—varying the thickness of the photo-active layer [31] or the use of optical spacers to control the micro-cavity effects [32] . However, the strong blue–green fullerene absorption prevents the design of a single-mode red or NIR cavity. Harrison et al. [33] have shown that a narrow response can be obtained around the absorption onset of neat MEH-PPV thick photodiodes via enhanced exciton dissociation efficiency at lower energies. In our current work, we introduce the new concept of charge collection narrowing (CCN) in thick bulk heterojunctions to achieve narrowband OPDs. The CCN devices operate based on narrowing the charge collection efficiency to the desired spectral region to overcome the above-mentioned limitations. We thus report the first sub-100 nm FWHM, visible-blind red and NIR photodetectors. Furthermore, the use of thick junctions markedly decreases the defect density [34] and therefore significantly suppresses the dark current [35] , resulting in high specific detectivities (~10 12 Jones) and a large linear dynamic range (LDR)- in this case 8 orders of magnitude. Moreover, we demonstrate that these CCN OPDs can be spectrally fine-tuned over a range of ~100 nm. This methodology is generic and the detection window can be chosen depending on the absorption onset of the junction materials. Spectral shape of the EQE OPDs utilizing thick junctions have previously been reported [15] , [22] , [33] , [35] . In particular, Armin et al. [35] recently described photodiodes with impressive performance metrics for broadband visible, IR-blind light detection using the archetypal bulk heterojunction organic semiconductor donor:acceptor blend of PCDTBT:PC70BM [(poly[ N -9″-heptadecanyl-2,7-carbazole- alt -5,5-(4′,7′-di-2-thienyl-2′,1′,3′-benzothiadiazole)]:PC70BM]. The quantum efficiency of these broadband devices was spectrally flat because efficient ‘volume generated’ charge carrier collection was achieved for all visible band wavelengths. In the current work, we utilize a completely different junction thickness regime (>1.5 μm) in combination with the CCN concept to produce the aforementioned narrowband spectral responses. It is important to note that our red narrowband devices utilize the same donor:acceptor combination (PCDTBT:PC70BM) as the broadband devices of Armin et al [35] . This shows that CCN is a device physics-related concept that delivers a new way of controlling spectral response over-and-above that afforded by the optical properties of the junction materials. As will be described later, the overall effect is to shape the internal quantum efficiency (IQE) to obtain spectral selectivity by markedly misbalancing the charge carrier transport. This is in stark contrast to any previously reported thick junction OPDs. To understand the CCN concept, we begin with the definition of the EQE which is generally given by [36] : Where, η abs is the light absorption within the photo-active layer (the heterojunction), η gen is the charge carrier generation quantum yield via exciton and CT state dissociation, and η coll is the photo-generated charge carrier collection efficiency. The IQE is the ratio of the EQE to the number of absorbed photons and can be spectrally flat in conventional photodiodes as shown in recent studies [21] , [29] . This means that the IQE does not influence the spectral sensitivity unless there are additional energy-dependent phenomena operating such as hot excitons [37] or marked differences in the Channel I and Channel II charge generation efficiencies [38] . Conventional thin film bulk heterojunction OPDs The working principles of conventional thin film bulk heterojunction and CCN OPDs are presented schematically in Fig. 1a–d , which show the device structure, photo-generated carrier distribution profile, and the EQE and absorption spectra of the photo-active layers, respectively. Although the figures are schematics for illustrative purposes, knowledge of the optical constants ( n and k see Methods) of all layers in the diode structure allows one to accurately simulate the actual optical field distributions, EQE and absorption using a transfer matrix analysis [29] , [39] , [40] . In this case the PCDTBT:PC70BM optical constants are used to demonstrate the concept. 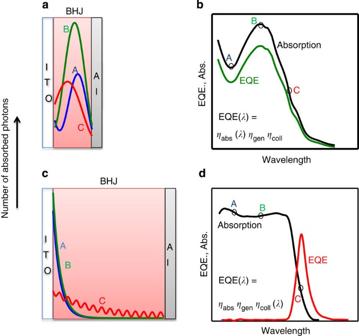Figure 1: Working principles of conventional and CCN OPDs. The photodiode structures are shown with the absorbed photon distribution for selected wavelengths marked on the absorption spectra within the active layer (A,BandC). Conventional narrowband OPD (a) and (b): in this case, photo-excitations are distributed within the active layer volume for all three wavelengthsA,BandC. The spectral behaviour of the EQE then follows the absorption spectrum within the active layer modified by any cavity interference effects. Charge collection-narrowed OPD (c,d): using a thick bulk heterojunction photo-active layer, shorter wavelength photons (AandB) are absorbed near the indium tin oxide (ITO) side, therefore the extraction of photo-generated electrons is hindered. In this case, the charge collection efficiency,ηcoll, is spectrally narrowed to only the wavelengths that are near the onset of the absorption (C) where the junction extinction coefficient is low. The EQE therefore peaks sharply at the onset of the absorption. Figure 1: Working principles of conventional and CCN OPDs. The photodiode structures are shown with the absorbed photon distribution for selected wavelengths marked on the absorption spectra within the active layer ( A , B and C ). Conventional narrowband OPD ( a ) and ( b ): in this case, photo-excitations are distributed within the active layer volume for all three wavelengths A , B and C . The spectral behaviour of the EQE then follows the absorption spectrum within the active layer modified by any cavity interference effects. Charge collection-narrowed OPD ( c , d ): using a thick bulk heterojunction photo-active layer, shorter wavelength photons ( A and B ) are absorbed near the indium tin oxide (ITO) side, therefore the extraction of photo-generated electrons is hindered. In this case, the charge collection efficiency, η coll , is spectrally narrowed to only the wavelengths that are near the onset of the absorption ( C ) where the junction extinction coefficient is low. The EQE therefore peaks sharply at the onset of the absorption. Full size image As shown in Fig. 1a , in a typical thin (~100 nm) junction OPD, the shape of the optical field distributions derived from the absorbed photons are somewhat independent of the incident light wavelength (for example, A , B and C ). In this figure, A and B are wavelengths above the optical gap, while C is near the absorption edge of the blend [21] . All three wavelengths produce volume photo-carrier generation, and, given the ‘thinness’ of the junction, one would not expect any significant spectral dependence of the charge carrier collection efficiency, η coll , since the drift distances for carriers generated at the three variable wavelengths are approximately the same. This feature of volume photo-carrier generation in thin junctions has been confirmed by spectral and field independent IQE and charge photogeneration measurements in thin junctions [41] , [42] . In the absence of any exotic energy dependence of charge generation and transport, the EQE spectrum follows the spectral shape of the light absorption within the active layer. Therefore, one method to achieve a narrowband spectral response is to use narrowband absorbing organic semiconductors in a carefully designed junction (cavity) structure [30] . Charge collection-narrowed OPDs Figure 1c,d shows a thick junction equivalent of Fig. 1a,b . In this case, the heterojunction is chosen to be much thicker than the inverse of the absorption coefficient ( α ) of the photo-active layer, that is, it has a large optical density ( αd ≫ 1). Since α can typically be of order 10 5 cm −1 for organic semiconductor combinations, a photo-active layer thickness of ~2 μm will satisfy this condition. Under such circumstances, wavelengths A and B above the optical gap are very strongly absorbed and produce an exponential photo-carrier distribution profile according to the Beer–Lambert Law. There are no interference effects since no light reaches the back electrode, and one observes surface photo-carrier generation near the semi-transparent electrode. However, for light absorption at wavelengths near the optical gap ( C ), light can penetrate through the photo-active layer and volume photo-carrier generation occurs with the associated influence of optical interference. Consider now the relative charge collection efficiencies for the two cases, that is, the surface generation near the anode (responsible for hole extraction in reverse bias) for A and B (above-gap) wavelengths and volume generation for C (near-or-sub gap). When electrons and holes are photo-generated close to the anode as for A and B (the hole-extracting electrode, usually ITO), charge carrier drift preferentially extracts holes with short transit times [41] . Electrons must traverse the entire thick junction and therefore have much longer transit times. The diode displays strongly imbalanced charge carrier transport and negative space charge accumulates near the anode as a result of delayed electron extraction [43] . The space charge screens the electric field responsible for extracting the carriers (including holes). Consequently electrons and holes recombine and charge carrier collection is suppressed. This behaviour is akin to a shallow Schottky diode comprising a p -type semiconductor—the electric field is screened near the high work function electrode (ITO) in a direct analogy with the recombination (field free) zone in Schottky diodes [44] . The situation is very different for volume photogeneration ( C ) where the transport is more balanced. In a perfectly balanced diode, electrons and holes are extracted with the same efficiency preventing the formation of space charge. Hence, for wavelengths near the absorption onset, the collection efficiency is high, and for shorter wavelengths it is poor (in the limit zero) although a portion of photo-generated carriers (at C ) can also be lost due to the charge recombination near the anode. This imposes a strong wavelength dependence on the collection efficiency, which dominates the EQE as shown in Fig. 1d . The peak wavelength (and bandwidth) of the EQE can then be fine-tuned by adjusting the junction thickness as will now be demonstrated. We call this concept charge collection narrowing (CCN). By increasing the reverse bias voltage, the charge carrier transit time becomes shorter and that in turn decreases the formation of space charges for surface generated carriers. This causes the spectral selectivity to diminish at large reverse bias operating voltages. This is shown in Supplementary Fig. 1 . It is important to emphasize that these CCN OPDs can deliver high responsivity, low noise and sufficient speed at reverse bias voltages <2 V, where the narrowband spectral response is conserved. Low operating voltages are of course favoured because they deliver circuit simplicity and low power consumption. This sensitivity to the applied voltage re-affirms the basic concept of CCN. It is important to note that the thicknesses required for achieving the CCN-derived narrowband responses (microns) are much larger than those previously used for broadband organic semiconductor photodetectors (700 nm) that can still be considered as electrically thin [35] . The transport and optical properties of typical organic semiconductor donor:acceptor blends enable the large thicknesses used in CCN OPDs to guarantee surface charge generation for wavelengths outside the desired spectral range and volume charge generation for the required wavelengths. This vital condition is demonstrated by way of optical simulations in Supplementary Fig. 2 , which compares the charge generation distribution profiles in 700- and 2,000-nm thick PCDTBT:PC70BM junctions. Experimental results PCDTBT:PC70BM and poly[2,5-(2-octyldodecyl)-3,6-diketopyrrolopyrrole- alt -5,5-(2,5-di(thien-2-yl)thieno[3,2-b]thiophene)] (DPP-DTT):PC70BM BHJ systems were used to construct the CCN OPDs. These materials are archetypal high efficiency donor:acceptor combinations in organic photovoltaics [45] with their molecular structures shown in Fig. 2 . Both donor polymers when blended with PC70BM are broadband light absorbers and DPP-DTT has recently been introduced as a high mobility polymer for field effect transistors [46] . The PCDTBT:PC70BM heterojunction has an absorption onset at ~650 nm and DPP-DTT is a narrow optical-gap polymer with an absorption edge at ~950 nm ( Fig. 3a ). Using high molecular weight polymers ( M w =122 kDa, polydispersity index (PDI)=5.4 for PCDTBT and M w =350 kDa, PDI=2.8 for DPP-DTT) and appropriate solution thermal treatments, high solution viscosities enable the fabrication of thick, uniform films by spin coating [47] . Based on the thick junction methodology described above and an understanding of how to further suppress the dark current with hole-and-electron-blocking layers [35] , [48] , we arrived at the following optimized CNN, thick junction OPD structures: NIR OPD—ITO 80 nm/PEDOT:PSS 20 nm/DPP-DTT:PC70BM 2 μm/C60 50 nm/Al 100 nm and Red OPD—ITO 80 nm/PEDOT:PSS 20 nm/PCDTBT:PC70BM 2 μm/C60 50 nm/Al 100 nm. The normalized absorption spectra for the two blend systems (thin films on glass) and the normalized EQE of the OPDs are shown in Fig. 3a . Figure 3b shows the corresponding responsivity spectra (measured at −1 V). 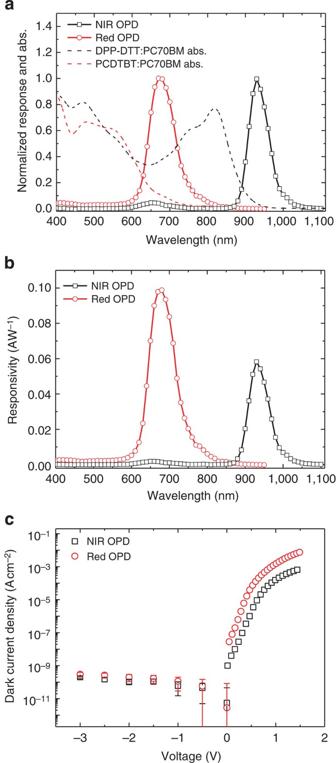Figure 3: Spectral dark current density-voltage response of the CCN red and NIR OPDs. (a) The normalized EQE of the narrowband CCN OPDs comprising thick junctions of PCDTBT (red) and DPP-DTT (NIR) blended with PC70BM. The normalized absorption of PCDTBT:PC70BM and DPP-DTT:PC70BM blends are also shown (dashed lines). The photoresponse peaks at the absorption edge as predicted under the CCN regime. (b) The responsivity of the OPDs under reverse bias voltage of 1 V. (c) Dark current density-voltage (J–V) curves for the CCN OPDs of (a) and (b). In forward bias, the dark current is measured by a normalJ–Vsweep but in reverse bias the extremely low dark current, means a time average of the current is taken for all points and the standard deviation (s.d.) of the fluctuations is specified by the error bars. 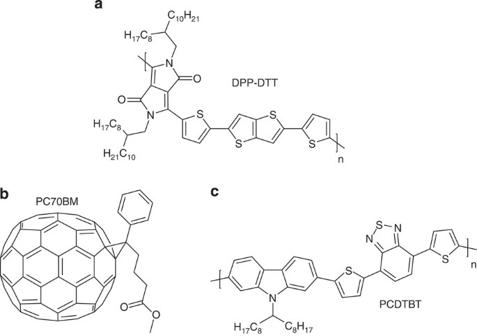Both red and NIR CCN OPDs have FWHM<90 nm. Figure 2: Molecular structures of the semiconductors used in this work. (a) DPP-DTT (electron donor) (b) PC70BM (electron acceptor) and (c) PCDTBT (electron donor). Figure 2: Molecular structures of the semiconductors used in this work. ( a ) DPP-DTT (electron donor) ( b ) PC70BM (electron acceptor) and ( c ) PCDTBT (electron donor). Full size image Figure 3: Spectral dark current density-voltage response of the CCN red and NIR OPDs. ( a ) The normalized EQE of the narrowband CCN OPDs comprising thick junctions of PCDTBT (red) and DPP-DTT (NIR) blended with PC70BM. The normalized absorption of PCDTBT:PC70BM and DPP-DTT:PC70BM blends are also shown (dashed lines). The photoresponse peaks at the absorption edge as predicted under the CCN regime. ( b ) The responsivity of the OPDs under reverse bias voltage of 1 V. ( c ) Dark current density-voltage ( J–V ) curves for the CCN OPDs of ( a ) and ( b ). In forward bias, the dark current is measured by a normal J–V sweep but in reverse bias the extremely low dark current, means a time average of the current is taken for all points and the standard deviation (s.d.) of the fluctuations is specified by the error bars. Full size image The dark current of OPDs under reverse bias theoretically depends on the electronics of the system [49] . However, the large density of defects (surface roughness, particles and ITO spikes) in solution-processed organic semiconductor junctions normally dominates the dark current, particularly in large area devices [34] . Use of a thick junction markedly decreases the defect density [35] . Figure 3c shows the dark current of the two CCN OPDs. In both cases, the dark current (under reverse bias) is extremely low, for example, at an operating reverse bias voltage of 1 V the dark currents are <10 −10 A. Although the dark current ( i d ) is an indicator of the noise figure of merit for photodetectors, one cannot directly define the noise current and specific detectivity via shot noise, which is proportional to the square root of the dark current [50] . In fact, the inferred shot noise, which is due to fluctuations in the Poissonian distributed quanta of the current (that is, electrons) obtained from the dark current , where e is the unit charge and B is the detection bandwidth (inversely proportional to the detection time constant), has been shown to differ from the real, measured noise even when the thermal noise is negligible [17] , [19] , [51] , [52] . If we use the shot noise to evaluate the noise equivalent power and the specific detectivity D * , we obtain a larger value for D * , of the order >10 13 Jones. However, by measuring the noise spectral density from the Fourier transform of the current versus time (see Supplementary Fig. 3 ), a more reliable value for the detectivity can be calculated from the noise power spectrum. In this case, the detectivity can be expressed as [34] : where λ is the detection wavelength, A the device area, h =Planck’s constant, c =speed of light and i noise the noise current spectral density (with unit of AHz −1/2 ). The i noise can be read from the noise spectrum at the detection frequency at which the EQE is measured (see Supplementary Fig. 3 ). 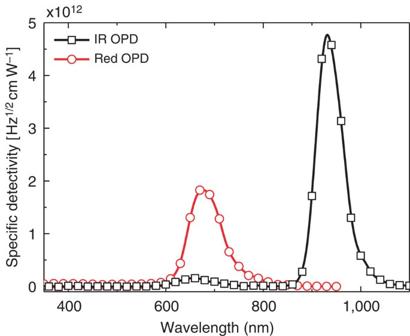Figure 4: Specific detectivity of red and NIR CCN OPDs. The specific detectivity is calculated based on the measured EQE (at 120 Hz) and the actual measured noise current under a reverse bias voltage of 1 V. Figure 4 shows the specific detectivities D * for the red and NIR CCN OPDs evaluated at 120 Hz, where the EQE was measured; these values are comparable within OPDs, whose specific detectivities range from between 10 9 to 10 12 at room temperature [2] , [53] . These results also demonstrate that our CCN OPDs are visible-blind, that is, there essentially is no contribution to the photocurrent from visible wavelengths. We note there is a minor contribution to the EQE and detectivity (<5%) at 650 nm in our NIR CCN OPDs due to a minimum in the DPP-DTT absorption at that wavelength. Figure 4: Specific detectivity of red and NIR CCN OPDs. The specific detectivity is calculated based on the measured EQE (at 120 Hz) and the actual measured noise current under a reverse bias voltage of 1 V. Full size image The LDR and frequency bandwidth are also critical performance parameters for photodiodes as they represent the light intensity operating range and temporal response of the device, respectively. For the red OPD, we observed 8 orders of magnitude linearity in the photoresponse (corresponding to either 80 dB or 160 dB following refs 51 , 52 , 54 and 2 [2] , respectively) and a −3 dB cut-off frequency of 100 kHz at −1 V ( Fig. 5 ). Due to light source limitations, we were not able to measure the frequency response and LDR for the NIR CCN OPD. However, because the charge carrier mobility of DPP-DTT is at least 3 orders of magnitude larger than PCDTBT [41] , [46] , one would expect an LDR and −3 dB frequency response at least as good as the PCDTBT:PC70BM devices. 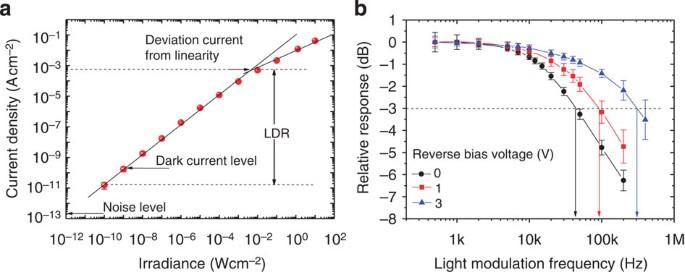Figure 5: Frequency and intensity response of the CCN red OPD. (a) Linear dynamic range (LDR) for the red OPD measured at −1 V (pump wavelength ~650 nm). The photodiode response is linear over 8 orders of magnitude. The error bars represent the s.d. from the mean value of six measurements. (b) Normalized response loss of the red OPD versus the input signal frequency (light modulation frequency at an intensity of ~1 mW cm−2). The −3 dB point is specified with the dashed line. The error bars correspond to the s.d. from the mean value of the signal versus time. Figure 5: Frequency and intensity response of the CCN red OPD. ( a ) Linear dynamic range (LDR) for the red OPD measured at −1 V (pump wavelength ~650 nm). The photodiode response is linear over 8 orders of magnitude. The error bars represent the s.d. from the mean value of six measurements. ( b ) Normalized response loss of the red OPD versus the input signal frequency (light modulation frequency at an intensity of ~1 mW cm −2 ). The −3 dB point is specified with the dashed line. The error bars correspond to the s.d. from the mean value of the signal versus time. Full size image Finally, and as indicated above, the peak EQE and hence the chosen spectral range of the CCN OPDs depends on the bulk heterojunction thickness. By increasing the junction thickness, wavelengths with only lower absorption cross-sections can penetrate to the cathode. Increasing the thickness thus causes longer wavelengths to contribute to surface charge carrier generation and this therefore shifts the response peak to longer wavelengths. In Fig. 6 , the EQE spectra for PCDTBT:PC70BM CCN OPDs with junction thicknesses of 1.5, 2 and 3 μm are shown as well as the absorption coefficient of the blend. The EQE can be fine-tuned over a 100 nm range through the absorption edge of the PCDTBT:PC70BM blend. It is however worth noting that the EQE does decrease as one tunes the spectral response towards the absorption edge of the blend. This arises due to less light absorption within the active layer relative to the parasitic absorption in the aluminium cathode ( Supplementary Fig. 4 ) as the wavelength increases. Further losses in CCN OPDs are associated with recombination of those charge carriers generated by the desired wavelengths near the anode ( Supplementary Fig. 2 ). However, it is important to note that the extraordinarily low dark current and noise of the thick junctions provide the possibility of amplification of photocurrent, which is then electronically manifested as a large specific detectivity. 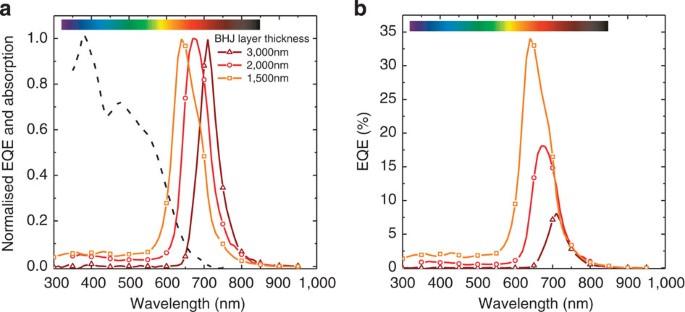Figure 6: The tunability of the CCN OPDs. The normalized EQE (a) and EQE (b) of PCDTBT:PC70BM photodiodes measured at 120 Hz and −1 V with different thicknesses allowing for fine-tuning the charge carrier photogeneration profile and thereby the EQE. As the active layer thickness increases from 1,500 to 3,000 nm the photogeneration in the volume occurs at longer wavelengths and the EQE peak red shifts from red to the NIR. The dashed line represents the absorption coefficient of the blend. Figure 6: The tunability of the CCN OPDs. The normalized EQE ( a ) and EQE ( b ) of PCDTBT:PC70BM photodiodes measured at 120 Hz and −1 V with different thicknesses allowing for fine-tuning the charge carrier photogeneration profile and thereby the EQE. As the active layer thickness increases from 1,500 to 3,000 nm the photogeneration in the volume occurs at longer wavelengths and the EQE peak red shifts from red to the NIR. The dashed line represents the absorption coefficient of the blend. Full size image In conclusion, we introduce the novel concept of CCN OPDs in a thick bulk heterojunction architecture. The CCN physics allows for precise tailoring of the spectral shape of the IQE. We demonstrate the first visible-blind sub-100 nm FWHM red and NIR photodetectors without the use of input filtering. The use of a thick junction decreases the defect density and therefore significantly suppresses the dark current resulting in high specific detectivities (~10 12 J) and LDR. Moreover, we demonstrate that these CCN OPDs can be spectrally fine-tuned by >100 nm. This methodology is generic and the detection window can be chosen depending on the absorption onset of the system. The wavelength selectivity of CCN narrowband OPDs is limited by the absorption onset of the donor and acceptor combination. If fullerenes are used, then the detection wavelengths possible using CCN are >600nm. Hence, to realize green and blue narrowband photodiodes wide optical-gap acceptors are required and this remains both a challenge and opportunity in the organic solar cell and photodiode community. Materials PCDTBT ( M w =122 kDa, PDI=5.4) was purchased from SJPC, Canada. The molecular weight of the PCDTBT was determined with gel permeation chromatography in 1,2,4-trichlorobenzene at 135 °C. PC70BM and C60 were purchased from American Dye Source Inc., Canada and used without further purification. DPP-DTT ( M w =350 kDa, PDI=2.8) was synthesized by the Institute of Materials Research and Engineering (IMRE) Singapore based on the methodology previously described [46] . Sample preparation The glass substrates with pre-etched ITO for bulk heterojunction OPDs were purchased from Kintec and mechanically cleaned by scrubbing using a soft cloth in a 90 °C warm Alconox (detergent) solution. Cleaning was followed by sequential ultrasonication in Alconox, de-ionized water, acetone and 2-propanol. After drying the substrates under a nitrogen flow, a 30-nm thick poly(3,4-ethylenedioxythiophene):poly(styrene sulfonate) (PEDOT:PSS; Baytron P VPAl4083) film was spin-coated at 5,000 r.p.m.. The PEDOT:PSS layer was baked at 170 °C for 10 min in air. All the device edges were cleaned with a wet cloth to prevent lateral current leakage through the PEDOT:PSS. Solutions of PCDTBT and DPP-DTT were prepared in 1,2-dichlorobenzene by stirring at 150 °C for an hour at a concentration of 10 mg ml −1 . Solutions were then slowly cooled to 80 °C and added to PC70BM in a weight ratio of 1:4 or 1:3 then stirred for 6 h at 80 °C. Solutions (at 80 °C) were then dispensed on the cold substrate. The fast cooling of the solution on dispensing on the cold surface results in a dramatic increase in the solution viscosity as shown by Wolfer et al. [47] The substrates were spun at 400 r.p.m. for >30 min followed by slow drying over 6 h at 40 °C. A 50 nm layer of C60 was deposited by thermal evaporation under a vacuum of ~10 −6 mbar followed by 100 nm of aluminium deposited under the same vacuum conditions to complete the devices. The resulting device areas were 0.2 cm 2 with six devices per substrate. EQE and optical simulations EQEs were measured using a PV Measurements Inc. QEX7 set-up at 120 Hz. The optical field distributions in the photodiodes were simulated using a computer code based on the transfer matrix method developed by van de Lagemaat and co-workers [44] from the National Renewable Energy Laboratory (NREL, USA). For these simulations optical constants (refractive index and extinction coefficients) of the all the materials in the structure are required. In this regard, we performed spectroscopic ellipsometry (SE) measurements for PCDTBT:PC70BM films on silicon wafers ( Supplementary Fig. 5 ; used for transfer matrix simulations in Fig. 1 ). Optical constants of the other layers have been measured previously [30] . The SE measurements were performed with a J.A. Woollam ultraviolet-variable angle spectroscopic ellipsometer (VUV-VASE; GEN II) with autoretarder. J.A. Woollam WVASE32 software was used to fit the data. Dark/photocurrent and LDR measurement Dark currents and photocurrents were measured using an Agilent semiconductor analyzer B1500A by averaging the current over time for each voltage step. The devices were mounted on an optical table in a Faraday cage with a small aperture for the laser beam. Triax leads were used to minimize the measurement noise. An ITO on glass panel that was electrically connected to the cage by silver paste to further reduce the electrical noise covered the aperture. A diode laser operating continuously at 650 nm (Laserver) was used as the illumination source with a series of neutral density filters purchased from Thorlabs and Holmarc for the LDR measurements. Temporal response Frequency dependent measurements were made using a Nichia red LED modulated by using an arbitrary wave generator (Agilent 33250A). The photocurrent response of the photodiode was recorded using a digital storage oscilloscope (LeCroy Waverunner A6200). How to cite this article: Armin, A. et al. Narrowband light detection via internal quantum efficiency manipulation of organic photodiodes. Nat. Commun. 6:6343 doi: 10.1038/ncomms7343 (2015).